Synaptobrevin2 is the v-SNARE required for cytotoxic T-lymphocyte lytic granule fusion Cytotoxic T lymphocytes kill virus-infected and tumorigenic target cells through the release of perforin and granzymes via fusion of lytic granules at the contact site, the immunological synapse. It has been postulated that this fusion process is mediated by non-neuronal members of the soluble N -ethylmaleimide-sensitive factor attachment protein receptor complex protein family. Here, using a synaptobrevin2-monomeric red fluorescence protein knock-in mouse we demonstrate that, surprisingly, the major neuronal v-SNARE synaptobrevin2 is expressed in cytotoxic T lymphocytes and exclusively localized on granzyme B-containing lytic granules. Cleavage of synaptobrevin2 by tetanus toxin or ablation of the synaptobrevin2 gene leads to a complete block of lytic granule exocytosis while leaving upstream events unaffected, identifying synaptobrevin2 as the v-SNARE responsible for the fusion of lytic granules at the immunological synapse. Cytotoxic T lymphocytes (CTLs) kill tumorigenic and/or virus-infected cells through release of lytic substances from secretory lysosomes, also called lytic granules (LGs). The release process is restricted to the contact area between CTL and target cell, the immunological synapse (IS). The formation of the IS is initiated by the interaction of surface CD3/T-cell receptor complexes with antigens presented by the target cell through MHC class I molecules. A complex intracellular signalling cascade results in the accumulation of proteins needed for LG fusion at the IS, most notably the LGs themselves. Before LGs are being transported along the cytoskeleton towards the IS, they undergo several maturation steps, trafficking through numerous intracellular compartments like early endosomes, late endosomes, multivesicular bodies and lysosomes. Most membrane fusion events in eukaryotic cells are mediated by the formation of the SNARE (soluble N -ethylmaleimide-sensitive factor attachment protein (SNAP) receptor) complex [1] , [2] . It consists of a four-helical bundle formed between a SNARE protein residing in the vesicle membrane (v-SNARE) and up to three SNARE proteins residing in the target membrane (t-SNARE) [3] . The SNARE complex possesses remarkable stability, as evidenced by its high melting point and resistance against detergents. The neuronal SNARE complex consisting of the v-SNARE synaptobrevin2 (also called VAMP2) and the t-SNAREs syntaxin1 and SNAP-25 is also the target of tetanus toxin and botulinum neurotoxins, which cleave individual amino acids of SNARE proteins and lead to a complete block of synaptic transmission, resulting in paralysis and death. The currently known 38 members of the mammalian SNARE family are not promiscuous in forming a SNARE complex, but rather possess a remarkable specificity for their cognate SNARE partners [4] . Once the specific SNARE complex is formed, the opposing membranes are pulled tightly together, enforcing the lipid fusion reaction [5] . In regulated exocytosis, accessory proteins like synaptotagmin and complexin are additionally being required to overcome the energy barrier for fusion. The discovery that mutations in the t-SNARE syntaxin11 leads to familial hemophagocytic lymphohistiocytosis type 4 (FHL4), a life-threatening immune disorder in humans, confirmed the speculation that SNARE proteins have an essential role in LG maturation and release [6] , [7] . Although a number of SNARE proteins have been shown to influence individual LG maturation steps [8] , [9] , [10] the molecular composition of the SNARE complex mediating the most important step of LG function, the final fusion with the plasma membrane to deliver the lethal hit that enables target cell killing, remains unknown. For the t-SNAREs several candidates have been proposed [7] , [11] , whereas no candidate v-SNARE protein has emerged so far. In this manuscript, we have investigated the localization of several v-SNARE candidates in resting and conjugated CTLs and demonstrate that only the major neuronal v-SNARE, synaptobrevin2, is localized to LGs at the IS. Interference with synaptobrevin2 function by gene ablation or tetanus toxin treatment leads to a complete block of LG fusion without affecting upstream maturation steps. Thus, we have identified synaptobrevin2 as the v-SNARE essentially required for mediating LG fusion in CTLs. Synaptobrevin2 is the only v-SNARE on LGs In an effort to identify candidate v-SNAREs for the fusion of LG with the plasma membrane we performed immunofluorescence studies with isoform-specific antibodies against different VAMP isoforms on mouse CTLs conjugated with target cells. One day before fixation, CTLs were transfected with a granzyme B-teal fluorescent protein (GzmB–TFP) fusion construct to specifically label LGs. We then performed structured-illumination microscopy (SIM) [12] to resolve a potential colocalization with a resolution of 100 nm in x , y and z -direction. As shown in Fig. 1 , VAMP3 (cellubrevin), VAMP4 and VAMP7 did not colocalize with granzyme B (Pearson’s coefficient ‘ r ’ of 0.05, 0.1 and 0.22, respectively), demonstrating that they are not localized on LG. In contrast, synaptobrevin2 (VAMP2) strongly colocalized with LG, indicated by a Pearson’s coefficient [13] of correlation of 0.62. As we have shown previously that VAMP8 is also not localized to LG [14] , these data demonstrate that synaptobrevin2 is the only v-SNARE that localizes to LGs at the IS in mouse CTL. 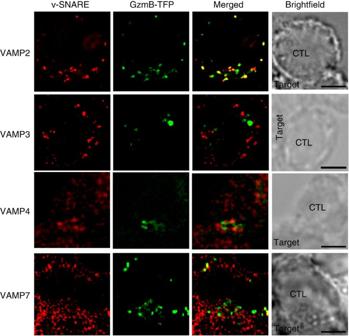Figure 1: Localization of individual v-SNAREs in activated CTLs from mouse. High-resolution SIM images (100 nm resolution inx,yandz) of mouse CTLs transfected with granzyme B-TFP (green channel, middle) and immunolabeled with antibodies against individual v-SNAREs (red channel, left). Overlay of both channels revealed that only VAMP2 (synaptobrevin2) colocalizes with the lytic granule marker granzyme B, whereas VAMP3 (cellubrevin), VAMP4 and VAMP7 were virtually absent from lytic granules. The corresponding Pearson’s coefficients for colocalization are given in the text. Scale bar, 2 μm. Figure 1: Localization of individual v-SNAREs in activated CTLs from mouse. High-resolution SIM images (100 nm resolution in x , y and z ) of mouse CTLs transfected with granzyme B-TFP (green channel, middle) and immunolabeled with antibodies against individual v-SNAREs (red channel, left). Overlay of both channels revealed that only VAMP2 (synaptobrevin2) colocalizes with the lytic granule marker granzyme B, whereas VAMP3 (cellubrevin), VAMP4 and VAMP7 were virtually absent from lytic granules. The corresponding Pearson’s coefficients for colocalization are given in the text. Scale bar, 2 μm. Full size image Synaptobrevin2-mRFP mice as a tool to study LG secretion We next sought to perform functional studies on the role of synaptobrevin2 in LG maturation and release. For that purpose, we selected a knock-in strategy in which the endogenous synaptobrevin2 was replaced by a synaptobrevin2-monomeric red fluorescence protein (Syb2-mRFP). As the Syb2-mRFP remained under the control of the endogenous synaptobrevin2 promotor, every naturally expressed synaptobrevin2 molecule in every tissue of the mouse would be labelled by the mRFP fluorophore. Homozygous Syb2-mRFP knock-in mice carrying an mRFP-cDNA instead of the stop codon in exon 5 of the synaptobrevin2 gene, followed by a neomycin resistance cassette in the 3′ untranslated region, were generated by homologous recombination in embryonic stem cells ( Supplementary Fig. S1a ). After removal of the neomycin cassette mice were bred to yield homozygous Syb2-mRFP offspring and backcrossed for 10 generations into C57/BL6. The Syb2-mRFP knock-in mice, which were routinely verified by genotyping ( Supplementary Fig. S1b ), were born at the expected Mendelian frequency. In contrast to the embryonically lethal synaptobrevin2 knockout mice [15] they showed no obvious behavioural or morphological defect. Western blot of brain homogenates demonstrated the expected 25–30 kDa shift in migration compared with endogenous Syb2 ( Supplementary Fig. S1c ). Importantly, the expression levels of Syb2 and Syb2-mRFP in the different mouse strains were comparable and no breakdown products were detectable. A gene dosage effect was detected for both Syb2 and Syb2-mRFP ( Supplementary Fig. S1c,d ). To rule out that the mRFP fused to the C-terminus interferes with the function of synaptobrevin2 we performed comprehensive morphological analysis and electrophysiological measurements from neurons and neuroendocrine cells, because in these cell types synaptobrevin2 is the major v-SNARE driving Ca 2+ -dependent fusion of synaptic vesicles [15] , [16] , [17] , [18] . The obtained results ( Supplementary Figs S2–S4 ) demonstrate that the addition of mRFP does neither alter the morphological and functional characteristics of central synapses in brain nor the hormone release from neuroendocrine cells. In conjunction with its inconspicuous phenotype we conclude that the Syb2-mRFP mouse is a suitable tool to study the localization and function of synaptobrevin2 in CTLs. Having established the full functionality of Syb2-mRFP in synaptic transmission from neurons and neuroendocrine cells we investigated the role of synaptobrevin2 in LG fusion from CTLs. Western blot analysis of purified CTLs (98.9% purity; Supplementary Fig. S5 ) using a monoclonal anti-synaptobrevin2 antibody revealed a single band of the expected molecular weight in both Syb2-mRFP and WT CTLs ( Fig. 2a ), indicating the expression of synaptobrevin2 in CTLs. To verify that Syb2-mRFP is, as wild-type synaptobrevin2 ( Fig. 1 ), specifically localized on LGs we transfected CTLs from Syb2-mRFP mice with GzmB–TFP and performed SIM [12] . SIM images of resting and conjugated cells, which formed an IS with their target cell, revealed an exclusive localization of synaptobrevin2 on LGs (Pearson’s coefficient [13] of correlation of 0.85; Fig. 2b ). We also performed correlative fluorescence electron microscopy (CLEM) [19] to confirm that the fluorescent puncta in CTLs from Syb2-mRFP mice are indeed LGs. As shown in Fig. 2c , the alignment of an 80-nm thick transmission electron micrograph with a serial 400 nm thick SIM image gave an almost perfect overlap of fluorescence with large dense-core structures typical for LGs. Finally, we also performed FACS-based assays to measure the surface expression of CD25 and CD107 to demonstrate the activation and LAMP1 degranulation capacity of CTLs, respectively, from Syb2-mRFP and WT control mice and found no significant difference between the two populations ( Supplementary Fig. S6a,b ). Therefore, CTLs from Syb2-mRFP mice show normal distribution and function. 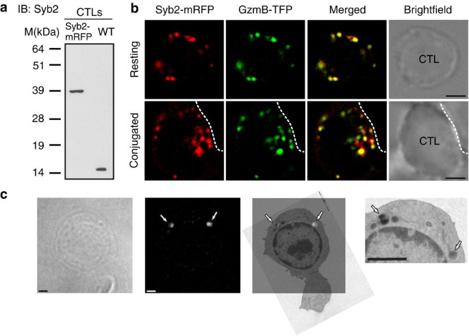Figure 2: Ultrastructure and function of CTLs from synaptobrevin2 knock-in mice. (a) Western blot detection of synaptobrevin2 in CTLs from WT and Syb2-mRFP mice using a monoclonal anti-synaptobrevin2 antibody. (b) Colocalization of synaptobrevin2 and granzyme B in CTLs from syb2-mRFP mice either having no contact with target cells (Resting; upper panel) or after incubation with target cells for 30 min (Conjugated; lower panel). Stippled white line indicates the border of the target cell membrane that is in contact with the CTL. The colocalization was quantified for 10 cells by Pearson’s coefficient ‘r’ (r=0.851). Scale bar, 2 μm. (c) Representative correlative fluorescence electron microscopy image of a resting CTL obtained from Syb2-mRFP mice. From left to right: Bright field image, processed SIM image, SIM/TEM overlay and magnification of TEM image. Arrows indicate synaptobrevin2-positive lytic granules. Scale bar, 1 μm for the two left images and 2 μm for the right image. Figure 2: Ultrastructure and function of CTLs from synaptobrevin2 knock-in mice. ( a ) Western blot detection of synaptobrevin2 in CTLs from WT and Syb2-mRFP mice using a monoclonal anti-synaptobrevin2 antibody. ( b ) Colocalization of synaptobrevin2 and granzyme B in CTLs from syb2-mRFP mice either having no contact with target cells (Resting; upper panel) or after incubation with target cells for 30 min (Conjugated; lower panel). Stippled white line indicates the border of the target cell membrane that is in contact with the CTL. The colocalization was quantified for 10 cells by Pearson’s coefficient ‘ r ’ ( r =0.851). Scale bar, 2 μm. ( c ) Representative correlative fluorescence electron microscopy image of a resting CTL obtained from Syb2-mRFP mice. From left to right: Bright field image, processed SIM image, SIM/TEM overlay and magnification of TEM image. Arrows indicate synaptobrevin2-positive lytic granules. Scale bar, 1 μm for the two left images and 2 μm for the right image. Full size image Tetanus toxin impairs degranulation We next used a degranulation assay to test whether synaptobrevin2 is involved in the fusion of lysosomes with the plasma membrane of CTLs. Transfection of CTLs with tetanus toxin light chain fused to GFP (GFP-TeNT-LC) resulted in a large reduction in degranulation in comparison with cells transfected with GFP alone ( Fig. 3a ). As tetanus toxin not only cleaves synaptobrevin2, but also its non-neuronal homologue cellubrevin (VAMP3) [20] , we performed a degranulation assay on CTLs isolated from cellubrevin knockout mice. In comparison with WT CTLs we observed no reduction in degranulation from cellubrevin-deficient CTLs ( Fig. 3b ), indicating that the reduction in degranulation from tetanus toxin-treated CTLs was probably due to the cleavage of synaptobrevin2 rather than of cellubrevin. We confirmed this result in an assay independent of TeNT transfection by examining degranulation of E19 CTLs derived from synaptobrevin2 knockout mice. These synaptobrevin2-deficient CTLs showed, in comparison with CTLs derived from WT littermates, a dramatic reduction in degranulation ( Fig. 3c ). Thus, synaptobrevin2 is expressed in CTLs, localizes exclusively to LGs and is required for the fusion of lysosomal compartments with the plasma membrane. 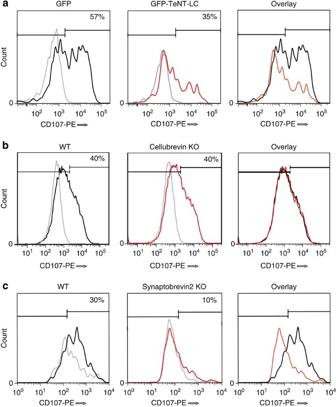Figure 3: Functional synaptobrevin2 is required for efficient degranulation of CTLs. (a) FACS-based degranulation assay in GFP (57%, left) and GFP-TeNT-LC (35%, middle) transfected CTLs using CD107-PE conjugated antibody. Overlay (right) of CD107-PE fluorescence in stimulated GFP- and TeNT-transfected cells illustrates the significant reduction in degranulation upon TeNT treatment. Light grey lines in left and middle are histograms from unstimulated control cells. Shown are representative histograms from four independent experiments. (b) FACS-based degranulation assay in WT (40%, left) and cellubrevin KO (40%, middle) CTLs using CD107-PE conjugated antibody. Overlay (right) of CD107-PE fluorescence in stimulated WT and cellubrevin KO CTLs verifies the lack of an effect on degranulation in the absence of cellubrevin. Light grey lines in left and middle are histograms from unstimulated control cells. Shown are representative histograms from four independent experiments. (c) FACS-based degranulation assay in WT (30%, left) and synaptobrevin2 KO (10%, middle) CTLs using CD107-PE conjugated antibody. Overlay (right) of the CD107-PE fluorescence in stimulated WT and synaptobrevin2 KO CTLs shows the dramatic reduction in degranulation in the absence of synaptobrevin2. Light grey lines in left and middle are histograms from unstimulated control cells. Shown are representative histograms from two independent experiments. Figure 3: Functional synaptobrevin2 is required for efficient degranulation of CTLs. ( a ) FACS-based degranulation assay in GFP (57%, left) and GFP-TeNT-LC (35%, middle) transfected CTLs using CD107-PE conjugated antibody. Overlay (right) of CD107-PE fluorescence in stimulated GFP- and TeNT-transfected cells illustrates the significant reduction in degranulation upon TeNT treatment. Light grey lines in left and middle are histograms from unstimulated control cells. Shown are representative histograms from four independent experiments. ( b ) FACS-based degranulation assay in WT (40%, left) and cellubrevin KO (40%, middle) CTLs using CD107-PE conjugated antibody. Overlay (right) of CD107-PE fluorescence in stimulated WT and cellubrevin KO CTLs verifies the lack of an effect on degranulation in the absence of cellubrevin. Light grey lines in left and middle are histograms from unstimulated control cells. Shown are representative histograms from four independent experiments. ( c ) FACS-based degranulation assay in WT (30%, left) and synaptobrevin2 KO (10%, middle) CTLs using CD107-PE conjugated antibody. Overlay (right) of the CD107-PE fluorescence in stimulated WT and synaptobrevin2 KO CTLs shows the dramatic reduction in degranulation in the absence of synaptobrevin2. Light grey lines in left and middle are histograms from unstimulated control cells. Shown are representative histograms from two independent experiments. Full size image Synaptobrevin2 cleavage abolishes LG fusion In principle, interference with any maturation step preceding fusion could also result in the observed reduction in degranulation upon TeNT treatment or in synaptobrevin2-deficient CTLs. To rule out this possibility and to visualize fusion of LGs in real-time we performed total internal reflection fluorescence microscopy (TIRFM). CTLs from Syb2-mRFP mice were allowed to settle on anti-CD3/anti-CD28-coated coverslips upon which they immediately formed an IS as indicated by the accumulation of LG in the TIRF plane [9] . The average number of LGs over the entire observation period (120 s at 10 Hz) was indistinguishable between TeNT-treated and control CTLs ( n =10; Fig. 4a ), demonstrating that synaptobrevin2 cleavage did not interfere with any LG maturation step upstream of docking at the IS membrane. In agreement with previous TIRFM data from adrenal chromaffin cells [21] , [22] , the average dwell time of LGs at the plasma membrane was significantly reduced in TeNT-treated CTLs to 37.2±7.0 s ( n =27) when compared with control CTLs where the average dwell time was 84.8±19.4 s ( n =27; Fig. 4c ). Most importantly, the fusion of LGs with the plasma membrane, which we regularly observed in control CTLs (five fusion events from 14 cells from three experiments; Fig. 4b and Supplementary Movie 1 ), was entirely abolished in all TeNT-treated CTLs (13 cells from three experiments) ( Fig. 4d ). These data identify synaptobrevin2 as the v-SNARE required to mediate the final step of cytolytic function of T lymphocytes, the fusion of LGs to deliver the lethal hit on target cells. 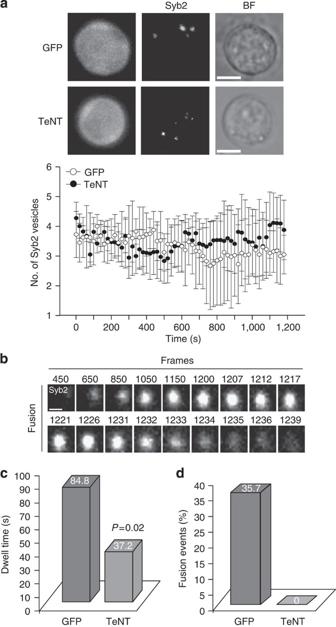Figure 4: Synaptobrevin2 is required for fusion of lytic granules at the IS (a) (Top) Epifluorescence (left), TIRFM (middle) and bright field (right) images depicting the number of synaptobrevin2-containing vesicles in GFP and GFP-TeNT-LC transfected CTLs for a single frame. Scale bar, 2 μm. (Bottom) Quantification of the number of synaptobrevin2-containing vesicles over time (acquisition frequency: 10 Hz) in GFP and GFP-TeNT-LC transfected CTLs. Error bars represent s.d. (b) Representative TIRFM images showing the fusion of a synaptobrevin2-containing vesicle in real-time. The vesicle arrived at the IS at frame 650 and fused with the plasma membrane at frame 1233. The acquisition frequency was 10 Hz. (c) Dwell time of synaptobrevin2-containing vesicles in TIRFM in GFP-TeNT-LC and GFP transfected CTLs. The average dwell time of synaptobrevin2-containing vesicles in GFP-TeNT-LC cells was 37.2±7.0 s and 84.8±19.4 s in GFP cells (P=0.02). (d) Percentage of LG fusion events in GFP (n=14) or GFP-TeNT-LC (n=13) transfected CTLs. Figure 4: Synaptobrevin2 is required for fusion of lytic granules at the IS ( a ) (Top) Epifluorescence (left), TIRFM (middle) and bright field (right) images depicting the number of synaptobrevin2-containing vesicles in GFP and GFP-TeNT-LC transfected CTLs for a single frame. Scale bar, 2 μm. (Bottom) Quantification of the number of synaptobrevin2-containing vesicles over time (acquisition frequency: 10 Hz) in GFP and GFP-TeNT-LC transfected CTLs. Error bars represent s.d. ( b ) Representative TIRFM images showing the fusion of a synaptobrevin2-containing vesicle in real-time. The vesicle arrived at the IS at frame 650 and fused with the plasma membrane at frame 1233. The acquisition frequency was 10 Hz. ( c ) Dwell time of synaptobrevin2-containing vesicles in TIRFM in GFP-TeNT-LC and GFP transfected CTLs. The average dwell time of synaptobrevin2-containing vesicles in GFP-TeNT-LC cells was 37.2±7.0 s and 84.8±19.4 s in GFP cells ( P =0.02). ( d ) Percentage of LG fusion events in GFP ( n =14) or GFP-TeNT-LC ( n =13) transfected CTLs. Full size image We show here that synaptobrevin2 (VAMP2) is expressed in CTLs where it exclusively localizes to LGs. By taking advantage of a new synaptobrevin2-mRFP knock-in mouse we demonstrate that synaptobrevin2 functions as a v-SNARE to mediate the fusion of LGs with the plasma membrane, the most important molecular event in CTL function. The discovery of gene mutations in patients with severe immune disorders like FHL generated a high interest in the molecular mechanisms of LG biogenesis, maturation and fusion in CTLs, CD4 helper cells and natural killer cells [11] , [23] , [24] . It became apparent that most disease-causing proteins possess isoforms that have an important role in synaptic transmission from neurons and neuroendocrine cells [11] , [23] , [25] . As the molecular mechanisms leading to synaptic transmission have been studied in great detail [26] , [27] , it was assumed that, for example, syntaxin11, the defective protein in FHL4, functions as a t-SNARE mediating the fusion of LGs with the plasma membrane [23] . However, SNARE complexes function in a large variety of intracellular membrane fusion reactions [1] , [2] . In CTLs, LGs traffic from the trans-Golgi network through early endosomes, late endosomes, multivesicular bodies and lysosomes before becoming a mature, fusogenic LG. Interruption at any step of this maturation process through defective SNARE proteins would lead to a reduction of CD107 surface expression in a FACS-based degranulation assay, the mostly used secretion assay in the field. Similar results would be obtained in Cr 51 and granzyme B release assays, two other established methods to investigate CTL function. Indeed, such an effect has been described in CTLs from mice deficient in vti1b and VAMP8, two SNARE proteins involved in endosomal trafficking of immature LG [28] . Therefore, based on the current literature [29] , [30] it is unclear whether syntaxin11 indeed serves as a t-SNARE to mediate the LG fusion reaction or whether it mediates earlier maturation steps. On the basis of a recent expression and localization study in human CTLs [14] numerous other potential t-SNARE candidates do exist, namely syntaxin3, syntaxin4, syntaxin6, syntaxin8, syntaxin13, syntaxin16 and syntaxin17. It is evident from this large number that only functional studies in conjunction with high-resolution microscopy techniques like CLEM and TIRFM will enable the identification of the partner t-SNAREs for synaptobrevin2. The identification of synaptobrevin2 as the v-SNARE required for LG fusion with the plasma membrane is somewhat surprising since neither syntaxin1 nor SNAP-25, the two other components of the neuronal SNARE complex mediating synaptic transmission, are expressed in CTLs [14] . Thus, other t-SNAREs must interact with synaptobrevin2 in CTLs to form a ternary SNARE complex mediating LG fusion. Besides the above-mentioned syntaxin isoforms SNAP-23 appears to be an excellent candidate, as its affinity to synaptobrevin2 in vitro is comparable to SNAP-25 (ref. 4 ). Also, it should be noted that the affinity of SNARE proteins to its partners is regulated by phosphorylation and leads to a different pool size of releasable granules [31] , [32] . As phosphorylation is a well known regulator of IS formation and function, it is plausible that CTLs regulate SNARE protein affinities dynamically depending on the physiological state. Furthermore, although release at neuronal synapses is optimized for speed, the release at the IS is rather optimized for accuracy. Therefore, it is probable that these synapses use different SNARE complexes for their respective fusion reactions. Synaptobrevin2 has also not been implemented as a candidate gene for immune diseases like FHL. This fact might be explained by the essential requirement of neuronal synaptic transmission for survival. Synaptobrevin2 knockout mice die immediately after birth, because they cannot breathe as a result of the loss of synaptic transmission in the Medulla oblongata and the brain stem [15] . Likewise, patients with defects in the synaptobrevin2 gene would die long before immune symptoms associated with FHL would begin to emerge. In conclusion, we have identified synaptobrevin2 as the v-SNARE mediating LG fusion at the IS of CTLs. The availability of the synaptobrevin2-mRFP knock-in mouse with their endogenously labelled LG will facilitate the identification of the t-SNAREs that form a SNARE complex with synaptobrevin2 to mediate the lethal hit of CTLs, the release of lytic substances from LGs at the IS. Generation of synaptobrevin2 knock-in mice and genotyping The targeting vector for the generation of synaptobrevin2-mRFP knock-in mice was constructed from of a 9-kb Hind III fragment containing the synaptobrevin2 locus, that was isolated from BAC-clone 48G12 of the RPCI-22 genomic mouse library ( www.bacpac.chori.org ) and subcloned into pSP73 (Promega, Madison, WI, USA). In the targeting vector, the stop codon in the last coding exon (Exon 5) of the synaptobrevin2 gene was replaced in-frame by the coding region for mRFP (kindly provided by R Tsien) using PCR with engineered primers and subcloning. Synaptobrevin2 was fused to mRFP via a soluble 9 aa linker (GGSGGSGGT) to prevent steric hindrance. A cassette containing the neomycin resistance gene under control of the CMV promoter and the Cre-recombinase gene under control of a testis specific promoter flanked by two loxP sites from plasmid pACN (kindly provided by M. Capecchi) was inserted downstream of the mRFP STOP codon. One copy of the HSV (herpes simplex virus) thymidine kinase gene was attached at the 3′-end of the targeting vector (see Fig. 2 ). Mice carrying the mutated synaptobrevin2-mRFP gene (m n /+) were generated by homologous recombination in embryonic stem cells (SV/129 R1) [33] as described previously [34] , [35] and identified by Southern blotting or PCR. The deletion of neomycin-Cre cassette after transmission through male germline was verified by PCR. The resulting mouse strain was backcrossed into C57/BL6 for 10 generations. Standard genotyping of homo- and heterozygous mice was done on lysed ear punches using primers 1+2 (1: 5′-CCTCATCATCATCATCGGTG-3′; 2: 5′-GGGCAGACTCCTCAGGGAT-3′). Cloning Plasmids coding for GFP-TeNT-LC and granzyme B-TFP were generated using standard cloning procedures. GFP-TeNT-LC: the synthetic tetanus light chain gene (Genbank accession number L19522.1 (ref. 36 ) (kindly provided by T. Binz (Medizinische Hochschule Hannover, Germany)) was subcloned in-frame of EGFP in pEGFP-C1 using Eco RI and Hind III sites. GzmB–TFP: plasmid pmTFP-N1 was generated by exchanging EGFP of pEGFP-N1 with mTFP1 (Allele Biotech, San Diego, CA, USA). Mouse GzmB was amplified by PCR from clone I730011M19 (ImaGenes, Berlin, Germany) to remove the stop codon and to generate a 5′- Hind III and 3′- Kpn I site and was inserted into pmTFP-N1. Cell isolation and antibodies Retina: freshly dissected mouse eyes were flash-frozen in liquid nitrogen-cooled isopentane. From the frozen mouse eyes, 10 μm-thick cryostat sections were cut, air-dried for 10 min and processed for immunolabeling with the indicated antibodies as previously described [37] . Hippocampal neurons were isolated as described previously [38] . Chromaffin cells were isolated as described previously [39] , [40] . Mouse CD8 T cells were obtained from spleen by commercially available CD8 isolation kits (Invitrogen). The isolated, naïve CD8 T cells were stimulated with anti-CD3/anti-CD28 activator beads (Invitrogen) and supplemented with recombinant IL-2 (50 U ml −1 ; BD Biosciences) for 3 days before being used for experiments. The anti-synaptobrevin2 antibody (Cl 69.1), anti-cellubrevin antibody (Cl TG 21.3) and anti-synaptophysin antibody (Cl 7.2) were kind gifts from R. Jahn (Max-Planck-Institute for biophysical chemistry, Göttingen, Germany). All other antibodies were from commercial sources (anti-VAMP4: aa 1–117, Synaptic Systems; anti-VAMP7: aa 10–177, Synaptic Systems; anti-RFP: M155-3, Cl 8D6, MBL International Corporation; anti-GAPDH: 14C10, Cell Signalling Technology; anti-CD3: 145-2C11, BD Pharmingen; anti-CD28: Cl 37.51, BD Pharmingen; PE and FITC anti-CD8a: 53-6.7, BD Pharmingen; FITC anti-CD25: Cl 7D4, BD Pharmingen; PE anti-CD107: 1D4B; BD Pharmingen; PE anti-IgG2a: α Isotype; BD Pharmingen). Electrophysiological Recordings The methods used for electrophysiological recordings of hippocampal neurons [38] , [41] and chromaffin cells [40] , [42] were previously described. Immunofluorescence Activated mouse CD8 T cells and P815 target cells were allowed to incubate for 30 min in the presence of anti-CD3 antibody (0.02 mg ml −1 ) to form an IS. Cells were fixed in ice cold 4% PFA in DPBS (Invitrogen) and stained with various antibodies. Structured-Illumination Microscopy The setup used was a prototype from Zeiss (Jena, Germany). Images were taken with a X63 Plan-Apochromat (NA 1.4) with excitation light of 488, 561 and 635 nm wavelengths and then processed for SIM to obtain higher resolutions. z-stacks of 200 nm step size were used to scan the entire cell. Zen 2009 software was used for acquisition and processing of the images for higher resolution. ImageJ v3.3 (Rasband, WS, USA National Institutes of Health, Bethesda, MD, USA) with the plugin JACoP [43] based on Pearson’s coefficient correlation factor ‘ r ’ was used for analysing colocalization. Correlative fluorescence electron microscopy Isolated mouse CD8 + cells of a synaptobrevin2-mRFP knock-in mouse were plated onto polyornithin (0.1 mg ml −1 )/CD11 (neutralizing antibody, 1:20) coated sapphire discs. The cells were allowed to settle for 20 min at RT. Sapphire discs were dipped into AIMV with 50% FCS, transferred into flat specimen carriers and frozen in a high-pressure freezing system (Leica EM PACT2/RTS). All samples were further processed in an automatic freeze-substitution apparatus (Leica AFS2). The carriers with the frozen specimens were cryo-transferred into dry flat embedding moulds inside the precooled (−140 °C) freeze-substitution chamber of the AFS2. The temperature was increased from −140 to −90 °C for 2 h. Cryosubstitution was performed at −90 to −70 °C for 21 h in anhydrous acetone and at −70 to −60 °C for 21 h with 0.3% (w/v) uranyl acetate in anhydrous acetone. At −60 °C the samples were infiltrated with increased concentrations (30, 60 and 100%; 1 h each) of Lowicryl (3:1 K11M/HM20 mixture with 0.3% uranyl acetate [44] . After 5 h of 100% Lowicryl infiltration, samples were UV polymerized at −60 °C for 24 h and for an additional 15 h while raising the temperature linearly to 5 °C. The samples were then kept at 4 °C until further processing at RT. After removing the sapphire discs the block face was trimmed for better orientation of the sections in structured-illumination and electron microscopes. Using the same diamond knife, cells were cut parallel to the sapphire so that a single 80 nm ultrathin section was serially followed by a 400-nm thick section, using a Leica EM UC7. The 80 nm ultrathin section was collected on a pioloform-coated copper grid, stained with uranyl acetate and lead citrate, and analysed with a Philips Tecnai12 Biotwin electron microscope. The 400 nm section was air-dried on a glass slide for 1 h and later cover-slipped with mounting-medium and used within 24 h for structured-illumination microscopy. Several pairs of sections could be cut from the same block face. Four hundred nanometer sections were used for structured-illumination microscopy. Images were taken with a X63 Plan-Apochromat NA 1.52 oil immersion lens. First, a bright field overview image was made, so that the cells could be found again in the 80 nm section in the TEM image. Cells of interest were cropped and structured-illumination analysis was done using z-stacks of 0.097 nm step size with excitation light of 561 nm wavelength. Images were overlaid in Corel Draw and aligned using features present in both the TEM image and the bright field or fluorescence SIM image of the same cell [45] . The polygon function was used to mark the features of the cell of interest in the bright field picture and the SIM image. The EM image was then aligned using these features. Then the transparent SIM image is aligned to the underlying TEM image. This allowed us to assign fluorescent objects in SIM to organelles observed in TEM. Evanescent-wave imaging The TIRF setup was as described previously [22] with the following additions: a solid-state laser 85 YCA emitting at 561 nm (Melles Griot, Carlsbad, CA, USA), a dual-view camera splitter (Visitron, Puchheim, Germany) to separate the red and green channels, a Visichrome Monochromator (Visitron) to acquire images in epifluorescence. CTLs from Syb2-mRFP mice that were transfected with GFP-TeNT-LC or GFP were washed and resuspended in 50 μl IMDM medium and allowed to settle for 3–4 min on anti-CD3/anti-CD28-coated coverslips. The cells were then perfused with extracellular solution containing 10 mM Ca 2+ to optimize Ca 2+ influx during secretion. Transfected cells were imaged for 10 min by TIRFM at 561 nm. The acquisition speed was set to 10 Hz and the exposure time was 100 ms. Experiments were carried out at room temperature. The analysis of LG dwell time (normalized to footprint area of cells) and fusion was performed with ImageJ v3.3 as detailed in ref. 9 . Fusion was defined by a >50% drop in fluorescence within one frame, that is, 100 ms. FACS-based LAMP1 degranulation assay The LAMP1 degranulation assay was performed as described in ref. 28 with minor changes. Briefly, in this assay we used a pure population of CD8 T cells that were activated with anti-CD3/anti-CD28-coated beads for 3 days. The activated T cells were transfected with either GFP-TeNT-LC or GFP. Cells were used for the FACS-based assay within 10 h of transfection. Cells were washed and resuspended in fresh IMDM medium with Golgi-Stop (containing monensin, BD Biosciences) in the presence of PE conjugated anti-CD107a antibody (eBioscience). Afterwards, the cell suspensions were transferred to the wells coated with or without anti-CD3/anti-CD28 antibody (96-well plate) and incubated at 37 °C, 5% CO 2 for 4 h. Then the cells were washed, resuspended in FACS buffer (PBS/0.1%BSA/5% FCS) and evaluated by flow cytometry (BD Biosciences). Data were analysed using FlowJO. Gating was performed based on the negative control (no antibody). Degranulation was calculated as the percentage of cells that showed an increase in CD107a membrane fluorescence upon stimulation in contrast to the respective unstimulated counterparts. For the experiments with synaptobrevin2 KO and WT, E19 spleen cells were cultured in DMEM medium (Invitrogen) and stimulated with anti-CD3/anti-CD28-coated beads for 5 days and supplemented with 100 U ml −1 IL-2. CD8 T cells were labelled with anti-CD8 FITC antibody (BD Biosciences) and the degranulation assay was performed as described above. Statistical analysis Statistical differences between two sets of data were analysed with a Mann–Whitney U -test as specified in the figure legends. How to cite this article: Matti U. et al. Synaptobrevin2 is the v-SNARE required for cytotoxic T-lymphocyte lytic granule fusion. Nat. Commun. 4:1439 doi: 10.1038/ncomms2467 (2013).